A spontaneousCdt1mutation in 129 mouse strains reveals a regulatory domain restraining replication licensing Cdt1 is required for loading the replicative DNA helicase MCM2/7, a process known as DNA replication licensing. Here we show that 129 mouse strains express a Cdt1 mutated allele with enhanced licensing activity. The mutation, named Δ 6 PEST, involves a six-amino acid deletion within a previously uncharacterized PEST-like domain. Cdt1 Δ 6 PEST and more extensive deletions exhibit increased re-replication and transformation activities that are independent of the Geminin and E3 ligase pathways. This PEST domain negatively regulates cell cycle-dependent chromatin recruitment of Cdt1 in G2/M phases of the cell cycle. Mass spectrometry analysis indicates that Cdt1 is phosphorylated at sites within the deleted PEST domain during mitosis. This study reveals a conserved new regulatory Cdt1 domain crucial for proper DNA licensing activity and suggests a mechanism by which the presence of Cdt1 in G2/M phases does not lead to premature origin licensing. These results also question the usage of 129 mouse strains for knockout analyses. DNA replication is initiated at specific loci called replication origins [1] , [2] that are recognized by the origin recognition complex (ORC). This six-subunit complex is conserved in all eukaryotes and functions as an ATPase required for loading of the replicative helicase MCM2/7, thus allowing the formation of prereplication complexes (pre-RCs) [3] . Cdc6 and Cdt1 are two essential cofactors for pre-RC establishment, a process known as licensing [4] , [5] . Differently from other pre-RC components, Cdt1 does not display enzymatic activity and is believed to bridge together the ORC and MCM2/7 complexes during licensing [6] , [7] . Licensing is highly regulated to ensure that it occurs only once per cell cycle [4] . Inappropriate licensing (for instance, as a consequence of deregulated Cdt1 activity) leads to origin reactivation, re-replication, genomic stress and instability and, ultimately, to oncogenic transformation [5] , [8] , [9] , [10] . Cdt1 activity is controlled by several, partly redundant pathways. First, Geminin directly binds to Cdt1 and inhibits its licensing activity [11] , [12] . Cdt1 regulation also involves the ubiquitin proteasome pathway and at least three different E3 ligases, namely SCF Skp2 (refs 13 , 14 ), CRL4 Cdt2 (refs 15 , 16 ) and APC Cdh1 (ref. 17 ), depending on the cellular context. Finally, Cdt1 is also regulated at the chromatin level. Cdt1 binds to chromatin in a cell cycle-dependent fashion with high occupancy in G1 phase and low in mitosis [18] , [19] , [20] . It is not fully understood how this cell cycle-specific binding is controlled, but cyclin-dependent kinase (CDK) activities are involved in inhibiting Cdt1 association with chromatin [18] , [20] . Restraining Cdt1 binding to chromatin might impair licensing activity; however, the functional significance of the cell cycle-dependent chromatin association of Cdt1 is not well understood. While analysing DNA replication in mouse embryonic stem (ES) cells, we discovered a novel, spontaneous mutation of the Cdt1 gene that consists of a six-amino acid deletion within the previously uncharacterized PEST-like domain in the amino-terminal part of Cdt1 (Δ 6 PEST allele). Here we show that this PEST domain is important for repressing Cdt1 activity, independently of the Geminin and E3 ligase pathways. Specifically, the PEST domain is phosphorylated during mitosis and regulates the cell cycle-dependent association of Cdt1 with chromatin. The Cdt1 Δ 6 PEST allele could also have phenotypic implications, as it is specifically found in the 129/Sv strain that is widely used in knockout studies [21] . Identification of the Cdt1 Δ 6 PEST allele During a recent analysis of DNA replication in mouse pluripotent cells [22] , [23] , we characterized the expression of various replication factors. P19 (C3H/He strain) and CGR8 (129/Ola strain) cells were found to express similar amount of ORC2, MCM7, Cdt1 and proliferating cell nuclear antigen (PCNA) ( Fig. 1a ). As the Cdt1 form expressed in CGR8 ES cells was slightly smaller in size (arrowhead in Fig. 1a ), we sequenced the Cdt1 complementary DNA from both cell lines. P19 cells expressed a 557-amino-acid-long, ‘wild-type’ (WT) Cdt1 protein that was identical to the mouse Cdt1 homologue reported in many databases ( Fig. 1b and data not shown). Conversely, CGR8 cells expressed a 551-amino-acid-long Cdt1 with a small in-frame deletion in the N terminus ( Fig. 1b ) that caused the loss of exactly one copy of a duplicated 18-nucleotide sequence, which corresponds to the ‘SPPADP’ sequence (underlined in Fig. 1b ). PCR analysis using primers that border the deletion established that the mutation was within exon 2 of Cdt1 ( Fig. 1c ). The deletion was localized in a Cdt1 region, which is rich in acidic, serine, threonine and proline residues, and corresponds to a previously uncharacterized PEST-like domain (hereafter referred as to ‘PEST’) that we also detected in other Cdt1 homologues ( Supplementary Fig. S1 ) [10] , [24] , [25] . As the mutation induced an in-frame deletion of six residues within the PEST domain, this allele was named Δ 6 PEST. 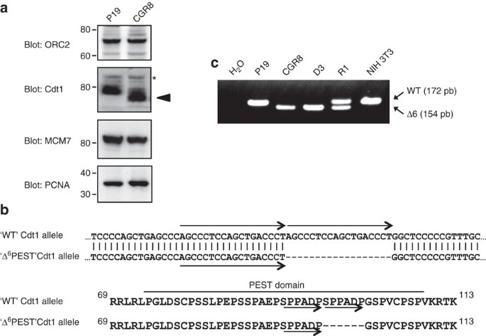Figure 1: Identification of the spontaneous Δ6PEST deletion mutant in the mouse 129 strains. (a) Lysates of exponentially growing mouse P19 and CGR8 cells were assessed by immunoblotting for expression of the indicated replication factors. The mutated form of Cdt1 expressed in the CGR8 ES cell line is indicated by an arrowhead. The asterisk indicates a non-specific band. (b) Cdt1 cDNA derived from CGR8 cells was cloned and sequenced. The homozygous mutation of Cdt1 consists in an 18-nucleotide deletion leading to a six-amino acid in-frame deletion within the PEST domain (Δ6PEST). The duplicated sequence found in the WT Cdt1 PEST domain is underlined. (c) PCR analysis of genomic DNA from P19, CGR8, D3, R1 and NIH 3T3 mouse cells using primers flanking the deleted region. PCR products corresponding to the WT and Δ6PEST (Δ6) alleles were separated on agarose gels. The size of the products is indicated. Figure 1: Identification of the spontaneous Δ 6 PEST deletion mutant in the mouse 129 strains. ( a ) Lysates of exponentially growing mouse P19 and CGR8 cells were assessed by immunoblotting for expression of the indicated replication factors. The mutated form of Cdt1 expressed in the CGR8 ES cell line is indicated by an arrowhead. The asterisk indicates a non-specific band. ( b ) Cdt1 cDNA derived from CGR8 cells was cloned and sequenced. The homozygous mutation of Cdt1 consists in an 18-nucleotide deletion leading to a six-amino acid in-frame deletion within the PEST domain (Δ 6 PEST). The duplicated sequence found in the WT Cdt1 PEST domain is underlined. ( c ) PCR analysis of genomic DNA from P19, CGR8, D3, R1 and NIH 3T3 mouse cells using primers flanking the deleted region. PCR products corresponding to the WT and Δ 6 PEST (Δ6) alleles were separated on agarose gels. The size of the products is indicated. Full size image We then evaluated the prevalence of the Cdt1 Δ 6 PEST allele and found that it was specifically present in the 129 mouse substrains ( Fig. 1c and Table 1 ). Indeed, 129/Sv, 129/Ola and 129/J mice were homozygous for the deleted allele, whereas all the other tested mouse strains were homozygous for WT Cdt1. Conversely, the R1 ES cell line, which is an F1 hybrid between 129/Sv and 129/SvJ [26] , was heterozygous for the allele ( Fig. 1c ). The presence in the 129/SvJ mice of a non-129 segment on chromosome 8, where lies the Cdt1 gene [27] , explains why the 129/SvJ strain express WT Cdt1 and not the Δ 6 PEST allele. As the 129/Sv, 129/J and 129/Ola strains were derived independently from the original 129 strain [27] , the original 129 strain might also contain the Cdt1 Δ 6 PEST allele. Table 1 Prevalence of the Δ 6 PEST allele in various mouse strains and the derived cell lines. Full size table Cdt1 licensing activity is under control of its PEST domain As PEST domains often are regulatory regions [28] , [29] , [30] , we investigated whether Cdt1 PEST domain affected licensing in vivo by using re-replication assays in U2OS cells. Re-replication was detected by flow cytometry as the proportion of transfected cells with >4n DNA content ( Supplementary Fig. S2 ). Similar to what was described for human CDT1 (refs 8 , 31 ), high expression of WT mouse Cdt1 (Cdt1:GFP ratio of 12:1) in U2OS cells induced re-replication ( Fig. 2a–c ). Interestingly, Cdt1 Δ 6 PEST displayed an enhanced re-replication activity in these assays ( Fig. 2a–c ). Moreover, Cdt1 variants in which both ‘SPPADP’ repeats (Δ 12 PEST) or the entire PEST domain (ΔPEST, Fig. 2a ) were deleted showed even stronger re-replication activity ( Fig. 2b ). When expressed at much lower levels (Cdt1:GFP ratio of 2:1), WT Cdt1 barely induced re-replication ( Fig. 2b ). Conversely, the ΔPEST mutant still exhibited strong re-replication, clearly illustrating the hyperactivity of this variant. In these experiments, all Cdt1 constructs were expressed at similar levels ( Fig. 2c ) and predominantly in the nucleus as indicated by immunofluorescence analysis ( Supplementary Fig. S3 ). 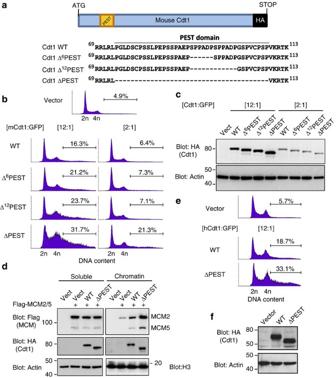Figure 2: Cdt1 licensing activity is negatively regulated by its PEST domainin vivo. (a) Constructs used in this study. (b) Re-replication assays showing the enhanced licensing activity of the Cdt1 PEST domain deletion mutants. U20S cells were cotransfected with the indicated mouse Cdt1 variants (mCdt1) and EGFP at the indicated ratios. Sixty hours post transfection, cells were processed and their DNA content analysed by flow cytometry. Transfected cells were gated based on the GFP signal. The percentage of re-replicating cells (>4n) is indicated. SeeSupplementary Figure S2for further details. (c) Expression of the Cdt1 variants in the U2OS cells analysed inbwas detected by immunoblotting. (d) Deletion of the PEST domain stimulates Cdt1 licensing activityin vivo. U20S cells were cotransfected with Flag-tagged MCM2 and MCM5, and Cdt1 variants (WT or ΔDDPEST), or empty vector (Vect) to monitor licensing in transfected cells exclusively. Protein levels in Triton-soluble and chromatin fractions were analysed by immunoblotting. (e) The regulatory role of the Cdt1 PEST domain is conserved. Re-replication assays of WT and ΔPEST human Cdt1 (hCdt1) were performed as inb. The percentage of re-replicating cells (>4n) is indicated. (f) Expression of Cdt1 corresponding to the experiment described ine. Figure 2: Cdt1 licensing activity is negatively regulated by its PEST domain in vivo . ( a ) Constructs used in this study. ( b ) Re-replication assays showing the enhanced licensing activity of the Cdt1 PEST domain deletion mutants. U20S cells were cotransfected with the indicated mouse Cdt1 variants (mCdt1) and EGFP at the indicated ratios. Sixty hours post transfection, cells were processed and their DNA content analysed by flow cytometry. Transfected cells were gated based on the GFP signal. The percentage of re-replicating cells (>4n) is indicated. See Supplementary Figure S2 for further details. ( c ) Expression of the Cdt1 variants in the U2OS cells analysed in b was detected by immunoblotting. ( d ) Deletion of the PEST domain stimulates Cdt1 licensing activity in vivo . U20S cells were cotransfected with Flag-tagged MCM2 and MCM5, and Cdt1 variants (WT or ΔDDPEST), or empty vector (Vect) to monitor licensing in transfected cells exclusively. Protein levels in Triton-soluble and chromatin fractions were analysed by immunoblotting. ( e ) The regulatory role of the Cdt1 PEST domain is conserved. Re-replication assays of WT and ΔPEST human Cdt1 (hCdt1) were performed as in b . The percentage of re-replicating cells (>4n) is indicated. ( f ) Expression of Cdt1 corresponding to the experiment described in e . Full size image To evaluate the mechanism underlying the abnormal licensing activity of the Cdt1 mutants, we analysed MCM2/7 loading onto chromatin. In this assay, low levels of Flag-tagged MCM2 and MCM5 were coexpressed with WT or ΔPEST Cdt1 to monitor licensing in transfected U2OS cells. Overexpression of WT Cdt1 stimulated chromatin recruitment of MCM2/5, as expected ( Fig. 2d ). ΔPEST Cdt1 exhibited a much stronger licensing activity ( Fig. 2d ), as observed in re-replication assays. Cdt1 directly interacts with the MCM2/7 complex via its carboxy terminal [32] , [33] . We thus tested whether the Cdt1 PEST domain stimulated licensing through enhanced MCM2/7 interaction. Coimmunoprecipitation experiments revealed that the PEST domain was not involved in the formation of the Cdt1–MCM2/7 complex ( Supplementary Fig. S4A ). Cdt1 homologues also possess a PEST-like domain in their N terminus (see alignment in Supplementary Fig. S1 ). We thus evaluated whether the Cdt1 PEST domain regulated the activity of the human isoform as well. Re-replication assays clearly showed that human CDT1 ΔPEST also exhibited enhanced activity ( Fig. 2e ). Altogether, these results indicate that the PEST domain has an important and conserved role in negatively regulating the licensing activity of Cdt1. Cdt1 PEST domain acts independently of Geminin and E3 ligases The coiled-coil protein Geminin strongly interacts with Cdt1 and inhibits its licensing activity [11] , [12] . The functional interaction between the PEST domain of Cdt1 and Geminin was tested in re-replication assays. Ectopic expression of Geminin alone resulted in strong G1 block, presumably caused by the lack of pre-RC formation ( Fig. 3a ). Moreover, Geminin could suppress re-replication induced not only by WT Cdt1, as expected, but also by the ΔPEST Cdt1 mutant ( Fig. 3a ). This result indicates that the PEST domain of Cdt1 is not required for Geminin-mediated suppression of origin licensing. In addition, cotransfected Geminin increased the expression of both WT and ΔPEST Cdt1 ( Fig. 3b ), indicating that by blocking origin licensing and S-phase entry Geminin indirectly inhibited DNA synthesis-coupled degradation [13] of both Cdt1 variants. Finally, coimmunoprecipitation experiments indicated that the PEST deletions did not affect the Cdt1–Geminin interaction ( Fig. 3c ). These results suggest that the PEST domain does not act through Geminin. Similarly, the PEST domain was not required for association of Cdt1 with HBO1, an acetyl transferase that positively regulates licensing [34] ( Supplementary Fig. S4B ). From these results, we conclude that the PEST domain has a crucial role in negatively regulating Cdt1 activity independently of its two major binding partners. 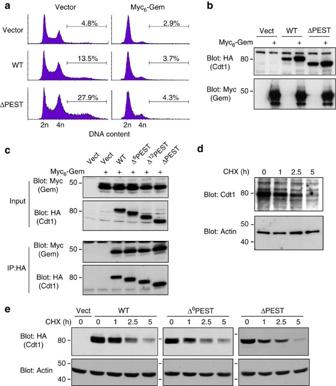Figure 3: The PEST domain regulates Cdt1 independently of Geminin and E3-ligase pathways. (a) Re-replication assays of WT and ΔPEST Cdt1 coexpressed with Geminin. The percentage of re-replicating cells (>4n) is indicated. (b) Expression of Cdt1 and Geminin corresponding to the experiment described ina. (c) U20S cells were cotransfected with Myc-tagged Geminin and the indicated HA-tagged Cdt1 variants. Forty-eight hours post transfection, lysates were immunoprecipitated with an anti-HA antibody. Proteins in the input lysates and immunoprecipitates were detected by immunoblotting. (d) Asynchronous U20S cells were treated with CHX (100 μg ml−1) for the indicated times. Expression of endogenous Cdt1 was analysed by immunoblotting. (e) The Cdt1 PEST mutants have similar half-lives. U20S cells were transfected with the indicated Cdt1 variants. Forty-eight hours post transfection, cells were treated with CHX as ind. Protein expression was monitored by immunoblotting. Figure 3: The PEST domain regulates Cdt1 independently of Geminin and E3-ligase pathways. ( a ) Re-replication assays of WT and ΔPEST Cdt1 coexpressed with Geminin. The percentage of re-replicating cells (>4n) is indicated. ( b ) Expression of Cdt1 and Geminin corresponding to the experiment described in a . ( c ) U20S cells were cotransfected with Myc-tagged Geminin and the indicated HA-tagged Cdt1 variants. Forty-eight hours post transfection, lysates were immunoprecipitated with an anti-HA antibody. Proteins in the input lysates and immunoprecipitates were detected by immunoblotting. ( d ) Asynchronous U20S cells were treated with CHX (100 μg ml −1 ) for the indicated times. Expression of endogenous Cdt1 was analysed by immunoblotting. ( e ) The Cdt1 PEST mutants have similar half-lives. U20S cells were transfected with the indicated Cdt1 variants. Forty-eight hours post transfection, cells were treated with CHX as in d . Protein expression was monitored by immunoblotting. Full size image The equivalent expression of all PEST mutants in transfected U2OS cells ( Fig. 2c ) suggests that the PEST domain does not regulate Cdt1 turnover. In asynchronous cells, endogenous Cdt1 had a half-life of ~1.5 h based on cycloheximide (CHX)-chase analysis ( Fig. 3d ). All Cdt1 PEST mutants had comparable degradation rates ( Fig. 3e ), confirming that the PEST domain was not involved in Cdt1 turnover. Nevertheless, we directly evaluated the possible implication of the PEST domain in the ubiquitin-mediated degradation of Cdt1 by its known E3 ligases, SCF Skp2 , CRL4 Cdt2 and APC Cdh1 . SCF Skp2 has an important role in regulating Cdt1 levels, notably in S phase [14] . Efficient association of Cdt1 with this ligase requires the presence of a cyclin-binding motif (RxL) and a CDK phosphorylation site (T29) on Cdt1 (ref. 35 ). Although both these sequences are localized outside the PEST domain, we investigated whether deletion within the PEST region could affect the accessibility to the degron. We first analysed the association of WT and ΔPEST Cdt1 with Cyclin A2 by immunoprecipitation experiments. Interaction of Cdt1 with Cyclin A2 did not require the PEST domain ( Supplementary Fig. S5A ). We then directly tested the sensitivity of the Cdt1 PEST variants to SCF Skp2 -dependent degradation in vivo . As previously observed [14] , overexpression of SKP2 (which ectopically activates SCF Skp2 ) downregulated WT Cdt1 expression ( Supplementary Fig. S5B ). Importantly, PEST deletion mutants were all similarly susceptible to SCF Skp2 -dependent degradation. These results indicate that the PEST domain is not involved in SKP2-mediated degradation of Cdt1. The CRL4 Cdt2 complex is a major and highly conserved E3 ligase that regulates Cdt1 proteolysis [36] . Perturbation of this pathway can induce strong re-replication and genomic instability [15] , [16] , [37] , illustrating its importance. Cdt1 contains a PCNA interacting protein motif (PIP) degron at its extreme N terminus. This sequence is involved in the interaction of Cdt1 with PCNA and the Cullin4 complex, leading to Cdt1 ubiquitinylation on chromatin and degradation [38] . We thus tested whether the PEST domain influenced the CRL4 Cdt2 -mediated degradation of Cdt1. First, the interaction of the Cdt1 PEST variants with PCNA was analysed by glutathione S -transferase (GST) pull-down assays. Recombinant PCNA specifically interacted with WT Cdt1 through the PIP degron ( Supplementary Fig. S5C ), confirming the specificity of this assay. In these conditions, the PEST domain deletion mutants could also associate with PCNA ( Supplementary Fig. S5D ). If Cdt1 modulation through the PEST domain and the PIP degron involves independent pathways, as suggested by the previous results, deletion of both regions should have an additive effect. We thus evaluated the activity of Cdt1 PIP degron and PEST domain mutants in vivo ( Supplementary Fig. S5E ) by performing re-replication assays after transfection of limiting amounts of Cdt1 variants to facilitate the detection of the stabilizing effect of the PIP degron mutation. As expected, deletion of the PIP degron (ΔPIP mutant) stabilized Cdt1 ( Supplementary Fig. S5F ) and strongly induced re-replication ( Supplementary Fig. S5G ), as previously reported [39] . In these conditions, WT Cdt1 barely induced re-replication ( Supplementary Fig. S5G , see also Fig. 2b ). Deletion of the PIP degron in the ΔPEST mutant (double ΔΔ mutant) also upregulated Cdt1 expression ( Supplementary Fig. S5F ) and its effect on re-replication was about double of what was observed with each single mutant ( Supplementary Fig. S5G ). These results indicate that the PIP and PEST regions regulate Cdt1 independently. A recent proteomic analysis revealed an unanticipated role of the E3 ligase APC Cdh1 in restraining Cdt1 activity [17] . D-boxes (the degrons recognized by this ligase) [40] in Cdt1 render the protein susceptible to Cdh1-mediated degradation. Cdt1 sequence analysis indicates that the PEST domain mutation should not alter the D-boxes and, therefore, that PEST mutant should be susceptible to APC Cdh1 degradation. Overexpression of Cdh1, which activates APC Cdh1 , downregulated WT Cdt1 expression ( Supplementary Fig. S5H ), as previously reported [17] . Cdh1 overexpression had a comparable effect also on ΔPEST Cdt1, indicating that the PEST domain does not influence APC Cdh1 -mediated degradation. Altogether, these results clearly show that the PEST domain of Cdt1 acts via a pathway that is independent of its known E3 ligases. PEST domain phosphorylation regulates Cdt1 chromatin loading Cdt1 displays cell cycle-dependent chromatin binding that is important for proper licensing regulation. As observed previously [18] , [19] , association of Cdt1 with chromatin was strong in NIH 3T3 cells synchronized in the G1 phase of the cell cycle, a period of pre-RC formation ( Fig. 4a ). Conversely, in S phase low expression of Cdt1 (caused by ubiquitin/proteasome-dependent degradation) resulted in very low chromatin association, thus preventing origin reactivation. Cdt1 started accumulating again in the G2 and M phases to prepare cells for the upcoming round of licensing during the next cell cycle. However, Cdt1 did not interact with chromatin during these phases ( Fig. 4a ) [18] , [20] , possibly to prevent illegitimate reinitiation of replication. In contrast, the ORC2 subunit of the ORC complex remained associated with chromatin throughout the cell cycle ( Fig. 4a ) [19] , [41] , highlighting the specific and regulated chromatin binding of Cdt1. As it is still unclear how Cdt1 is regulated at the chromatin level in higher eukaryotes, we asked whether the PEST domain was involved in this process. 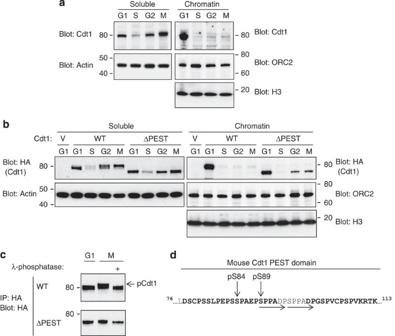Figure 4: Mitotic phosphorylation of the PEST domain regulates cell cycle-dependent Cdt1 chromatin association. (a) Cell cycle-dependent chromatin association of endogenous Cdt1 in mouse NIH 3T3 cells. Cells were synchronized in G1 (6 h release from quiescence), S (3 h release from a G1/S block), G2 (6 h release from G1/S block) and M (9 h release from G1/S block in presence of nocodazole, seeMethodsfor details) phases of the cell cycle. Expression of endogenous Cdt1 in the soluble and chromatin fractions was analysed by immunoblotting. (b) The PEST domain regulates Cdt1 association with chromatin during cell cycle progression. NIH 3T3 cells stably expressing physiological amounts of WT, ΔPEST Cdt1 or empty vector (V) were synchronized as ina. Expression of ectopic Cdt1 was monitored in soluble and chromatin fractions by immunoblotting. (c) HeLa S3 cells stably expressing HA-tagged mouse WT or ΔPEST Cdt1 were synchronized in mitosis (by nocodazole treatment) or in G1 phase (4 h release after mitotic shake-off). Ectopic Cdt1 was purified by immunoprecipitation and treated (+) with λ-phosphatase. The slower electrophoretic mobility of WT Cdt1 in mitosis is highlighted by an arrow. (d) HeLa S3 cells stably expressing tagged mouse Cdt1 were synchronized in mitosis. Ectopic proteins were purified by immunoprecipitation and phosphorylation site identification was done by MS analysis (seeMethodsfor details). Phosphorylation sites unambiguously identified within the Cdt1 PEST domain are indicated. Peptides observed by MS are highlighted in bold. Note that phospho-Ser89 lies in one of the ‘SPPADP’ repeats (underlined by arrows) deleted in 129 derived mouse strains. Figure 4: Mitotic phosphorylation of the PEST domain regulates cell cycle-dependent Cdt1 chromatin association. ( a ) Cell cycle-dependent chromatin association of endogenous Cdt1 in mouse NIH 3T3 cells. Cells were synchronized in G1 (6 h release from quiescence), S (3 h release from a G1/S block), G2 (6 h release from G1/S block) and M (9 h release from G1/S block in presence of nocodazole, see Methods for details) phases of the cell cycle. Expression of endogenous Cdt1 in the soluble and chromatin fractions was analysed by immunoblotting. ( b ) The PEST domain regulates Cdt1 association with chromatin during cell cycle progression. NIH 3T3 cells stably expressing physiological amounts of WT, ΔPEST Cdt1 or empty vector (V) were synchronized as in a . Expression of ectopic Cdt1 was monitored in soluble and chromatin fractions by immunoblotting. ( c ) HeLa S3 cells stably expressing HA-tagged mouse WT or ΔPEST Cdt1 were synchronized in mitosis (by nocodazole treatment) or in G1 phase (4 h release after mitotic shake-off). Ectopic Cdt1 was purified by immunoprecipitation and treated (+) with λ-phosphatase. The slower electrophoretic mobility of WT Cdt1 in mitosis is highlighted by an arrow. ( d ) HeLa S3 cells stably expressing tagged mouse Cdt1 were synchronized in mitosis. Ectopic proteins were purified by immunoprecipitation and phosphorylation site identification was done by MS analysis (see Methods for details). Phosphorylation sites unambiguously identified within the Cdt1 PEST domain are indicated. Peptides observed by MS are highlighted in bold. Note that phospho-Ser89 lies in one of the ‘SPPADP’ repeats (underlined by arrows) deleted in 129 derived mouse strains. Full size image To this aim, the WT Cdt1 and ΔPEST mutant were stably expressed in NIH 3T3 cells at low levels to ensure a near-physiological regulation of the exogenous protein ( Supplementary Fig. S6A ). Under these conditions, ectopic expression of Cdt1 did not perturb cell cycle progression ( Supplementary Fig. S6B ). As expected, binding of WT Cdt1 to chromatin was strong in cells in the G1 phase and barely detectable in cells in the S, G2 and M phases of the cell cycle ( Fig. 4b ; less than 5% of Cdt1 associated with chromatin in G1). Similarly, Cdt1 ΔPEST was strongly associated with chromatin in the G1 phase but not during the S phase, due to degradation of the protein ( Fig. 4b ). In the G2 and M phases, cells resynthesized Cdt1, as expected ( Fig. 4b , ‘soluble’). However, in contrast to WT Cdt1, Cdt1 ΔPEST partially reassociated with chromatin ( Fig. 4b , ~20% of Cdt1 bound to chromatin in G1 cells), strongly suggesting that the PEST domain has a role in regulating the cell cycle-dependent association of Cdt1 with chromatin. As previously reported [19] , [20] , Cdt1 displayed reduced electrophoretic mobility in mitotic cells ( Fig. 4a–c ). This shift was lost following phosphatase treatment ( Fig. 4c , upper panel), confirming that during mitosis Cdt1 is phosphorylated at unknown sites in mouse cells. Conversely, the mitotic shift was barely detected when using Cdt1 ΔPEST ( Fig. 4c , lower panel), suggesting that mitotic phosphorylation occurs within the PEST domain. Mass spectrometry (MS) analysis of mouse Cdt1 purified from mitotic cells clearly showed that the PEST domain of Cdt1 is phosphorylated on at least two sites in mitotic cells ( Fig. 4d , Supplementary Fig. S7 and Supplementary Table S1 ). Both Ser84 and Ser89 are targets of proline-directed kinases, such as CDKs. Importantly, the ‘SPPADP’ repeat (deleted in the 129/Sv mouse strain) was assigned unambiguously as phosphorylated. All together, these results support the hypothesis that phosphorylation of the PEST domain of Cdt1 in G2/M participates in limiting Cdt1 chromatin recruitment during mitosis, thus preventing inappropriate licensing. The PEST domain restrains oncogenic potential of Cdt1 Cdt1 can have oncogenic properties and is often overexpressed in human tumours [10] , [24] . To investigate whether the PEST domain regulates Cdt1 oncogenic potential, the transformation status of immortalized NIH 3T3 fibroblasts that stably overexpress Cdt1 ΔPEST or Δ 6 PEST ( Fig. 5a ) was evaluated using the foci formation and soft-agar growth assays. Although empty vector cells did not form foci or colonies in soft agar, WT Cdt1 overexpression favoured the formation of foci and stimulated, to some extent, cell growth in soft agar, confirming the oncogenic potential of Cdt1 ( Fig. 5b ). Overexpression of the PEST deletion mutants induced a much stronger transformation phenotype in both assays ( Fig. 5b ). We conclude that the PEST domain has a crucial role in restraining Cdt1 activity and that its deletion increases its transforming activity. 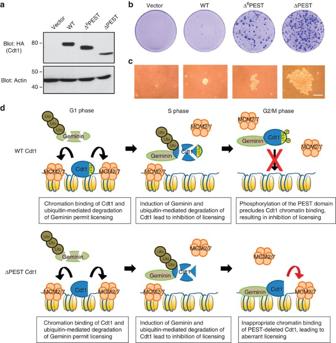Figure 5: The oncogenic potential of Cdt1 is negatively regulated by its PEST domain. (a) Stable expression of the different Cdt1 variants in NIH 3T3 cells. (b) Foci formation assay. The indicated stable NIH 3T3 cell lines were plated at similar density and cultured for 2–3 weeks without passaging. Cells were fixed and stained with crystal violet. Transformed cells that have lost the contact inhibition form densely stained foci. (c) Soft agar growth assay. The same stable NIH 3T3 cell lines were immobilized in soft agar and grown for 3–4 weeks. Proliferating colonies were visualized and counted by using a phase-contrast microscope. Shown are representative colonies. Scale bar, 50 μm. (d) Model of licensing control by Cdt1 PEST domain phosphorylation through regulation of Cdt1 association with chromatin. See Discussion for details. Figure 5: The oncogenic potential of Cdt1 is negatively regulated by its PEST domain. ( a ) Stable expression of the different Cdt1 variants in NIH 3T3 cells. ( b ) Foci formation assay. The indicated stable NIH 3T3 cell lines were plated at similar density and cultured for 2–3 weeks without passaging. Cells were fixed and stained with crystal violet. Transformed cells that have lost the contact inhibition form densely stained foci. ( c ) Soft agar growth assay. The same stable NIH 3T3 cell lines were immobilized in soft agar and grown for 3–4 weeks. Proliferating colonies were visualized and counted by using a phase-contrast microscope. Shown are representative colonies. Scale bar, 50 μm. ( d ) Model of licensing control by Cdt1 PEST domain phosphorylation through regulation of Cdt1 association with chromatin. See Discussion for details. Full size image The inbred 129/Sv mouse strain was the foundation for establishing ES cell cultures. It is still the most used strain for gene targeting in mice because the derived ES cells can be maintained in a pluripotent state and efficiently colonize the germ line [21] . Here we identified a spontaneous mutation in the Cdt1 gene that occurs specifically in 129 mouse substrains and show that the PEST domain (in which this mutation is localized) is involved in the control of replication licensing. The Δ 6 PEST allele corresponds to an in-frame deletion of one of two tandem ‘SPPADP’ repeat and displays elevated licensing and transforming activity. Interestingly, we show that the repeat is subjected to mitotic phosphorylation, suggesting that the enhanced licensing activity of Cdt1 Δ 6 PEST allele is due to impaired post-translational modification of the protein. Mice derived from the 129 strain are viable, indicating that the elevated Cdt1 licensing activity is mostly compensated. However, 129/Sv mice display specific phenotypic features, such as low fertility [42] , high incidence of testicular cancer (teratocarcinoma) [43] and pluripotency stability of the derived ES cells [21] . The elevated licensing activity caused by the PEST mutation could be implicated in some of these features. For instance, the Δ 6 PEST allele might predispose cells to tumorigenesis as a result of its intrinsic higher licensing activity, thus possibly explaining the higher tumour susceptibility of 129-derived mouse lines. Moreover, by favouring replication licensing, Δ 6 PEST Cdt1 could affect the replication origin repertoire as well as the chromatin organization and transcription [1] , [2] . As a consequence, this mutation might help in maintaining the stemness of 129/Sv-derived ES cells in culture. Cdt1 activity is regulated by multiple, overlapping regulatory pathways to control the G1–S progression, suggesting that it must be exquisitely adjusted to properly repress aberrant licensing and re-replication. Our results point to a crucial role of Cdt1 PEST domain phosphorylation in preventing illegitimate initiation of replication in G2/M phase (see model in Fig. 5d ). In the G1 phase, APC-dependent degradation of the licensing inhibitor Geminin allows Cdt1 to be active, leading to MCM2/7 complex loading on chromatin. In S phase, Cdt1 activity is restrained (to suppress re-replication) by Geminin protein stabilization and Cdt1 degradation coupled to DNA synthesis. In the G2/M phases, Cdt1 accumulates again, but cannot interact with chromatin because of the inhibitory activity of the phosphorylated PEST domain. In ΔPEST Cdt1-expressing cells, G1 and S phase events are expected to proceed normally. However, as cells reach the G2/M phases, ΔPEST Cdt1, which lacks key phosphorylation events, reassociates with chromatin, thus increasing the risk of aberrant licensing within the same cell cycle and consequently of re-replication. Phosphorylation of the Cdt1 PEST domain might directly inhibit its productive association with chromatin. Cdt1 recruitment to chromatin is dependent on the ORC complex but not on Cdc6, the other licensing factor [44] , [45] . In budding yeast, Cdt1 directly interacts with ORC6 (refs 6 , 46 ). Interestingly, CDK-dependent phosphorylation of ORC6 inhibits Cdt1/ORC association, thus preventing re-replication [47] . MS analysis revealed that the Cdt1 PEST phosphorylation sites are targets of proline-directed kinases, such as CDKs. As Cdt1 mitotic phosphorylation is CDK1-dependent [19] , [20] , it is tempting to implicate this kinase as the enzyme directly responsible for phosphorylation of the Cdt1 PEST domain. In vertebrates, Cdt1 homologues possess an N-terminal PEST-like region which displays some variability in both sequence and size. However, the PEST domain always possesses multiple putative CDK consensus sites (highlighted in Supplementary Fig. S1 ). In human cells, at least two of these proline-directed sites (Thr82 and Ser93) are phosphorylated in vivo [48] , [49] , suggesting that these phosphorylation sites are important conserved features of the Cdt1 PEST domain. Historically, PEST domains are acknowledged to be involved in protein degradation [10] , [24] , [25] . Although we cannot formally exclude that the Cdt1 PEST domain might control Cdt1 proteolysis in a short and specific period of the cell cycle, this study shows that Cdt1 degradation is mainly not regulated by its PEST domain. Accumulating evidences also show that PEST domain regions can regulate protein function through post-translational modifications [28] , [29] , suggesting different classes of PEST domains. For clarity, PEST sequence implicated in protein degradation could be referred as ‘PEST–degron’. On the other hand, the Cdt1 PEST domain described in this study could be referred as ‘Phospho-PEST’, as it is subject to evolutionarily conserved phosphorylation. In conclusion, we identified a Cdt1 PEST domain that is involved in the regulation of Cdt1 association with chromatin during the cell cycle. As mutations in this domain facilitate illegitimate re-replication and potentiate Cdt1 oncogenic properties, our data also suggest that the 129/Sv mouse strain, in which the Δ 6 PEST mutation occurs spontaneously, might not be the most suitable strain for targeting genes involved in cell cycle regulation or DNA metabolism. Cell culture and transfections U20S, HeLa S3, NIH 3T3, P19 and Platinum-E (Cell Biolabs) cells were grown in DMEM (Invitrogen) supplemented with 10% fetal bovine serum (FBS), 2 mM glutamine and antibiotics. The mouse ES cell line CGR8 (ref. 50 ) was cultured in Glasgow minimum essential medium supplemented with 10% FBS, 2 mM glutamine, 50 μM β-mercaptoethanol and 100 U ml −1 leukemia inhibitory factor (LIF). Cells were transfected using the Lipofectamine reagent (Invitrogen). For infection, viral particles were generated using Platinum-E ecotropic packaging cell line. HeLa S3 cells were transiently transfected with mouse Cationic Aminoacid Transporter 1 to render them susceptible to infection by ecotropic retroviruses. Puromycin (6 and 2.5 μg ml −1 ) were used to select S3 and NIH 3T3 cells, respectively. NIH 3T3 cells were synchronized by first rendering them quiescent (medium with 0.2% FBS, 24 h). Cells were then splitted in normal medium for 6 h (G1 phase) or in medium containing 2 mM thymidine for 18 h. Cells were then released from the G1/S block for 3 h (S phase), 6 h (G2 phase) or 9 h (M phase, in presence of 100 ng ml −1 nocodazole). HeLa S3 cells were synchronized as previously described [51] . Antibodies The anti-Cdt1 polyclonal antibody [1/1000] is an in-house antiserum raised against a C-terminal fragment of mouse Cdt1. Anti-Flag M2 [F1804; 1/1,000], anti-Actin [A5441; 1/5,000] and anti-PCNA [WH0005111M2; 1/2,500] monoclonal antibodies were from Sigma. The anti-Myc 9B11 monoclonal antibody [2276S; 1/1,000] was from Cell Signaling Technologies. The polyclonal anti-HA antibody [sc-805; 1/100] was from Santa-Cruz BioTechnologies. The anti-MCM7 [ab2360; 1/1,000] and histone H3 [ab1791; 1/2,500] antibodies were from Abcam. The anti-ORC2 antibody [1/1,000] was described previously [23] . Plasmid constructs Mouse Geminin, human CDT1 and human HBO1 cDNA were obtained from the IMAGE Consortium. Mouse WT and Δ 6 PEST Cdt1 were generated from P19 and CGR8 cell mRNA, respectively, by RT–PCR and cloned in pcDNA3-HAC terminal [51] . Mouse Cdt1 mutants (Δ 12 PEST, ΔPEST, ΔPIP and ΔΔ) were generated by PCR mutagenesis and cloned into pcDNA3-HAC terminal or pBabe-puro-HAC terminal. Human WT and ΔPEST CDT1 were obtained in a similar way. Myc-tagged Geminin and HBO1 were obtained by PCR amplification and cloned in pcDNA3-Myc 6 (ref. 52 ). GST fusion PCNA was produced using pHGST.1 (ref. 53 ). mCAT1 was amplified by RT–PCR from NIH 3T3 cells and cloned into pcDNA3. pBabe-puro [54] , Flag-Skp2 and -Cdh1, Myc-Cyclin A2 (ref. 51 ), HA-EGFP [55] and Flag-tagged MCM-2 and MCM-5 (ref. 56 ) constructs were previously described. Re-replication assay U20S cells were cotransfected with the tested constructs and an expression plasmid coding for EGFP. Sixty to seventy-two hours post-transfection, cells were trypsinized and fixed in 1% paraformaldehyde in PBS at room temperature for 15 min. Washed cells were fixed again in 70% ethanol in PBS and stored at −20 °C overnight. Cells were spun at 2,000 r.p.m. for 10 min, washed in PBS and treated with 50 μg ml −1 RNAse A. DNA was stained with 25 μg ml −1 propidium iodide. Cells were analysed with a FACSCalibur flow cytometer using the CellQuestPro software. Protein biochemistry Cell lysis, immunoprecipitation and western blotting were performed as described [51] . Briefly, cells were lysed in Triton lysis buffer (50 mM Tris–HCl pH 7.4; 100 mM NaCl; 50 mM NaF; 5 mM EDTA; 40 mM β-glycerophosphate; 1% Triton X-100 plus protease inhibitors cocktail) on ice for 30 min. The protein concentration of the clarified lysates was estimated using the bicinchoninic acid (BCA) method (Pierce). For immunoprecipitation experiments, equivalent amounts of protein samples were incubated at 4 °C with HA-coupled beads for 4 h. After extensive washing with Triton lysis buffer, bound proteins were eluted in boiling Laemmli buffer. For Cdt1/MCM coimmunoprecipitation, TK100 lysis buffer (20 mM Tris–HCl pH 7.9; 100 mM KCl, 5 mM MgCl 2 , 10% glycerol; 0.5% NP-40) was used [57] . Purification of GST fusion proteins was done as described previously [53] . GST pull-down assays were performed essentially as described [58] . Briefly, U20S cells transfected with various Cdt1 variants were lysed in GST-pd buffer (50 mM Tris-HCl pH 7.5; 150 mM NaCl; 1 mM EDTA; 10% glycerol; 0.5% NP-40 supplemented with protease inhibitors cocktail). Clarified lysates were incubated with 1 μg recombinant GST or PCNA–GST coupled to GSH beads at 4 °C for 2 h. After several washing steps in GST-pd buffer, proteins were eluted in boiling Laemmli buffer. For MS analysis of Cdt1 phosphorylation, ~40 *T150 Flask of mitotic HeLa S3 cells were used to purify stably expressed HA-tagged Cdt1 by immunoprecipitation. Chromatin isolation Chromatin and soluble fractions were obtained using the cytoskeleton (CSK) procedure [18] , [59] . Briefly, cells were lysed in CSK buffer (10 mM PIPES pH 6.8; 100 mM NaCl; 300 mM sucrose; 1 mM MgCl 2 ; 0.5 mM dithiothreitol; 0.2% Triton X-100; 1 mM ATP plus protease inhibitor cocktail) on ice for 10 min. Insoluble material was pelleted (3,000 r.p.m., 4 °C, 3 min). Supernatants (soluble fraction) were kept, while pellets were extracted a second time in CSK buffer. The final pellets (chromatin fraction) were solubilized in Laemmli buffer. Phosphatase assay HA-tagged WT or ΔPEST Cdt1 were purified by immunoprecipitation from HeLa S3 cells that stably express these proteins and were synchronized in G1 or M phases. The immunoprecipitates were washed with phosphatase buffer (50 mM HEPES pH 7.5, 100 mM NaCl, 2 mM dithiothreitol, 0.01% Brij 35). Dephosphorylation was performed using 200 U of λ-phosphatase (New England Biolabs) at 30 °C with agitation for 1 h. Reactions were stopped by addition of Laemmli buffer. Immunofluorescence U20S cells were plated on coverslips and transfected with the Cdt1 PEST variants. Twenty-four hours post transfection, cells were fixed in 3% paraformaldehyde in PBS and processed to detect HA-tagged Cdt1 as previously described [51] . DNA was visualized by DAPI (4',6-diamidino-2-phenylindole) staining. The subcellular localization pattern of the Cdt1 variants was analysed with a Leica DM6000 epifluorescence microscope. Images were acquired using a Coolsnap HQ CCD camera (Photometrics) and the Metamorph software (Molecular Devices). Protein half-life measurement Cdt1 turnover was determined by the CHX-chase method. Forty-eight hours after transfection with limiting amount of expression plasmids, U20S, P19 and NIH 3T3 cells were treated with 100 μg ml −1 of the translation inhibitor CHX (Sigma) for the indicated times. Total protein expression was monitored by western blotting. Cdt1 genotyping The Cdt1 PEST domain was genotyped using the following primers and PCR conditions: Cdt1PEST_F: 5′-TGTACTCTTTGTTCGCTTGACG-3′; Cdt1PEST_R: 5′-CTTCCCACCCCCAGTTTATT-3′; 94 °C, 30 s; 60 °C, 60 s; 72 °C, 45 s; 35 cycles. MS analysis To identify phosphorylation sites, about 200 ng Cdt1 purified from mitotic extracts were treated with trypsin (Promega) or AspN (Wako). After digestion, peptides were collected and analysed using a nanoESI LTQ_XL Orbitrap mass spectrometer (Thermo Fisher Scientific) coupled to an Ultimate 3000 HPLC (Dionex). A gradient of 0–40% B for 30 min and 80% B for 15 min (A=0.1% formic acid, 2% acetonitrile in water; B=0.1% formic acid in acetonitrile) at 300 nl min −1 was used to elute peptides from the capillary (0.075 mm × 150 mm) reverse-phase column (Pepmap, Dionex). Nano-ESI was performed with a spray voltage of 2.4 kV, heated capillary temperature of 200 °C and tube lens voltage of 140 V. A cycle of one full-scan mass spectrum (400–1,600 m/z ) at a resolution of 30,000, followed by five data-dependent MS/MS spectra was repeated continuously throughout the nanoLC separation. All MS/MS spectra were recorded using normalized collision energy and an isolation window of 2 m/z . Data were acquired using the Xcalibur software (v 2.0.7, Thermo Fisher Scientific). Data analysis was performed using MaxQuant 1.3.0.5 and standard parameters against the CPS_MOUSE database (November 2012). FDR was set at 1%. Foci formation assay Stable Cdt1 cell lines were plated in duplicate in 60 mm plates at equivalent density. Confluent cells were cultured for 2–3 weeks and the culture medium was changed every 2–3 days. Foci were stained with crystal violet dye. Soft agar growth assay Cells (10 5 ) for each stable Cdt1 cell line were mixed with medium supplemented with 0.4% agarose and placed on top of the 1% agarose layer. One millilitre medium was added to the solidified layer and changed every 2–3 days. After 3–4 weeks, colonies were counted in ten randomly selected fields using a phase-contrast microscope. How to cite this article: Coulombe, P. et al . A spontaneous Cdt1 mutation in 129 mouse strains reveals a regulatory domain restraining replication licensing. Nat. Commun. 4:2065 doi: 10.1038/ncomms3065 (2013).